Photocarrier relaxation pathway in two-dimensional semiconducting transition metal dichalcogenides Two-dimensional crystals of semiconducting transition metal dichalcogenides absorb a large fraction of incident photons in the visible frequencies despite being atomically thin. It has been suggested that the strong absorption is due to the parallel band or ‘band nesting’ effect and corresponding divergence in the joint density of states. Here, we use photoluminescence excitation spectroscopy to show that the band nesting in mono- and bilayer MX 2 (M=Mo, W and X=S, Se) results in excitation-dependent characteristic relaxation pathways of the photoexcited carriers. Our experimental and simulation results reveal that photoexcited electron–hole pairs in the nesting region spontaneously separate in k -space, relaxing towards immediate band extrema with opposite momentum. These effects imply that the loss of photocarriers due to direct exciton recombination is temporarily suppressed for excitation in resonance with band nesting. Our findings highlight the potential for efficient hot carrier collection using these materials as the absorbers in optoelectronic devices. Quasi-two-dimensional (2D) properties of layered transition metal dichalcogenides (TMDs) have long attracted interest in fundamental research [1] . Since the successful isolation of graphene and other atomically thin crystals from bulk layered compounds, renewed interest in the TMDs in their ultimate thickness regime led to the discovery of a range of their unique properties [2] , [3] , [4] . Recent findings on the novel optical properties of semiconducting 2D TMDs such as MoS 2 and WSe 2 include emerging band-gap photoluminescence (PL) [5] , [6] , controlled valley polarization [7] , [8] , [9] , strongly bound trions [10] , [11] , second harmonic generation [12] , [13] , strain-induced optical gap modulation [14] , [15] and surface sensitive luminescence [16] , [17] , [18] . Along with the attractive electrical properties [19] and recent progress in the materials synthesis [20] , [21] , these 2D TMDs show positive prospects for their applications in optoelectronic devices [22] , [23] . Individual layers of TMDs are excellent light absorbers despite being atomically thin [22] , [24] . Absorption spectra of MX 2 (M=Mo, W and X=S, Se) consist of characteristic peaks due to excitonic resonance and interband transitions. Recent ab initio studies have attributed the strong light-matter interaction to ‘band nesting’, which gives rise to singularity features in the joint density of states (JDOS) [25] . In the nesting region of the band structure, the conduction and valence bands are parallel to each other. The JDOS diverges for the resonance energy, resulting in giant enhancement in the corresponding optical conductivity. While singularities in the JDOS are present in common semiconductors and metals such as silicon and aluminium, divergence in optical conductivity due to band nesting is unique to low-dimensional systems [26] . The absorption is also enhanced for photon energies corresponding to transitions between van Hove singularity peaks in the DOS, which are attributed to heavy effective mass of carriers in MX 2 compounds [25] , [27] . Since absorption is highly efficient in the resonance conditions, understanding the resulting photocarrier relaxation dynamics is crucial in implementing these materials into light-harvesting devices. Photocarriers generated in the band-nesting region are of particular interest as the electrons and holes are expected to relax at the same rate, but with opposite momentum. In this work, we examine the relaxation processes of photoexcited carriers in mono- and bilayer MX 2 using photoluminescence excitation (PLE) spectroscopy and ab initio density functional theory (DFT) calculation. We show that the relaxation channel of the photoexcited carriers is strongly dependent on the excitation energy. Our findings reveal the unique implication of 2D band structure and the characteristic photocarrier relaxation. Strong light absorption Semiconducting group 6 TMDs consist of strongly bonded 2D X-M-X layers that are held together by weak van der Waals forces [1] , [27] . Each layer of M and X atoms forms a 2D hexagonal crystal ( Fig. 1a ). Monolayer MX 2 is noncentrosymmetric, while bilayer and bulk materials exhibit inversion symmetry [28] . The band gap is direct for monolayer MX 2 in contrast to the indirect gap of bilayer and thicker multilayers [5] , [6] . Since group 6 MX 2 is isoelectronic, general features of the electronic structure are similar. For monolayer MX 2 , the conduction band minimum and the valence band maximum are both located at the K/K′ point of the Brillouin zone ( Fig. 1b ) [29] , [30] , [31] , [32] , [33] . Conduction band valley at the Λ point and the valence band hill at the Γ point play a dominant role in the direct to indirect gap crossover. Band-nesting regions in Mo and W disulphide and diselenide monolayers occur midway between the Γ and Λ points [25] . 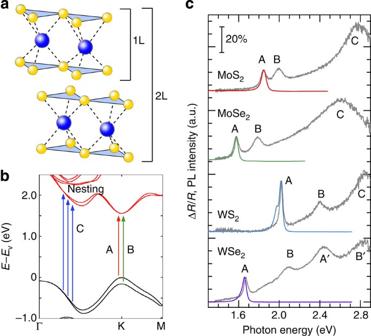Figure 1: Properties of monolayer MX2. (a) Lattice structures of monolayer and bilayer MX2. (b) The band structure of monolayer MoS2with the label of C calculated by the DFT. The arrows indicate the transition in A, B and the band nesting (C). (c) PL spectra (red, green, blue and purple curves) from excitation at the C (A' for WSe2) peak and differential reflectance spectra (grey curves) of monolayer MX2flakes on quartz substrates. The scale bar indicates 20% absorption based on the differential reflectance spectra. The PL intensity is normalized by the A exciton peak of the differential reflectance spectra for each material and the spectra are displaced along the vertical axis for clarity. Figure 1: Properties of monolayer MX 2 . ( a ) Lattice structures of monolayer and bilayer MX 2 . ( b ) The band structure of monolayer MoS 2 with the label of C calculated by the DFT. The arrows indicate the transition in A, B and the band nesting (C). ( c ) PL spectra (red, green, blue and purple curves) from excitation at the C (A' for WSe 2 ) peak and differential reflectance spectra (grey curves) of monolayer MX 2 flakes on quartz substrates. The scale bar indicates 20% absorption based on the differential reflectance spectra. The PL intensity is normalized by the A exciton peak of the differential reflectance spectra for each material and the spectra are displaced along the vertical axis for clarity. Full size image The optical signatures of the MX 2 materials reflect the basic features of the energy band structure. Figure 1c shows the PL and differential reflectance (Δ R / R ) spectra of monolayer MoS 2 , MoSe 2 , WS 2 and WSe 2 on a quartz substrate. The differential reflectance is an effective measure of the absorbance for ultrathin samples [34] . The resonance peaks A and B (labelled according to earlier conventions [33] ) correspond to excitonic transitions occurring at the K/K′ points of the k- space (See Fig. 1b ) [5] , [35] , [36] . Strong absorption at higher energies (C peak for MoS 2 , WS 2 and MoSe 2 ), which is estimated to be above 30% based on reflectance and transmittance measurements, arises from nearly-degenerate exciton states [37] . In a single-electron band structure picture, this feature corresponds to the region of the Brillouin zone where the valence and conduction bands are nested [25] . The absorption features of WSe 2 are typically more complex due to strong effects of the Se p orbitals [33] but the strong absorption above ~2.4 eV may be attributed partly to band nesting. The calculated band structure indicates that excited electrons and holes in the nesting region relax to their immediate band extremum. This corresponds to Λ valley and Γ hill for electrons and holes, respectively. The intraband relaxation is known to be extremely fast (<500 fs) in mono- and few-layer MoS 2 and dominates other relaxation processes [38] , [39] , [40] (see more information in Supplementary Table 1 ). Radiative recombination of the electron–hole pairs separated in the k -space requires emission or absorption of a phonon and is a slow process, typically resulting in low yield emission. The carrier lifetime in the indirect emission process can be estimated to be on the order of 1 ns based on previous studies [38] , [41] . On the other hand, direct excitons exhibit lifetime on the order of 100 ps with correspondingly higher quantum yield (QY) [38] . Here, we investigate the effect of band nesting on the behaviour of photoexcited electron–hole pairs in monolayer MX 2 by studying their excitation-dependent PL QY. To obtain micro-PLE spectra from micrometer-sized flakes of mechanically exfoliated samples, we utilized a super-continuum light source coupled to a tunable laser filter as the excitation source (see Methods for details). The excitation power was kept constant and low to avoid undesired nonlinear effects. 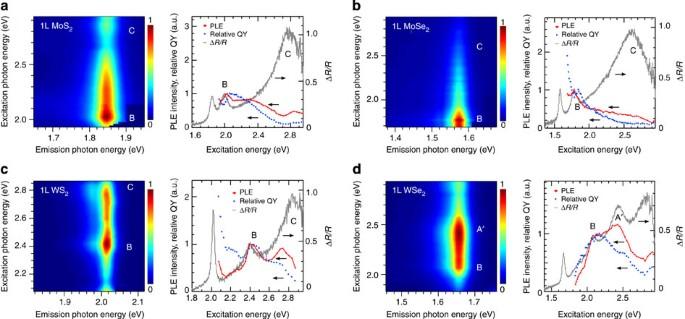Figure 2: PLE spectra of monolayer MX2. PLE intensity map (left panel), PLE spectra and relative QY of emission (right panel) for band gap emission for monolayer (a) MoS2, (b) MoSe2, (c) WS2and (d) WSe2flakes. Differential reflectance spectra are also shown for comparison. The PLE spectra are based on the integrated intensity of the A peak in the PL spectra at each excitation energy. Each PLE spectrum is normalized by the B exciton peak of each material. Effect of band nesting Figure 2 shows the PLE intensity map of monolayer (a) MoS 2 , (b) MoSe 2 , (c) WS 2 and (d) WSe 2 flakes and comparisons between the PLE spectra (red plots), relative QY of emission (blue dots) and the differential reflectance spectra (grey lines). The relative QY is estimated by dividing the integrated PL intensity by the absorption at the excitation energy. It can be seen that the PLE intensity is enhanced when the excitation is in resonance with the B exciton absorption. In contrast, for MoS 2 and MoSe 2 , the PLE intensity at the C absorption peak is suppressed or only weakly enhanced. We note that similar suppression of the PLE is seen for WS 2 and WSe 2 for excitation near the C and B′ absorption peaks, respectively. In all cases, the relative QY drops consistently for excitation energies above the B peak resonance. We attribute this behaviour to the spontaneous separation of electron–hole pairs in the k -space due to band nesting. Figure 2: PLE spectra of monolayer MX 2 . PLE intensity map (left panel), PLE spectra and relative QY of emission (right panel) for band gap emission for monolayer ( a ) MoS 2 , ( b ) MoSe 2 , ( c ) WS 2 and ( d ) WSe 2 flakes. Differential reflectance spectra are also shown for comparison. The PLE spectra are based on the integrated intensity of the A peak in the PL spectra at each excitation energy. Each PLE spectrum is normalized by the B exciton peak of each material. Full size image To further verify this effect, we studied the PLE spectra of bilayer MoS 2 ( Fig. 3a ). The absorption features of bilayer samples are similar to those of monolayers, exhibiting excitonic resonance peaks A and B and strong C peak absorption due to band nesting ( Fig. 3b ). According to our previous studies [32] , [34] , bilayer MoS 2 and WS 2 exhibit indirect band gap emission involving Λ valley in the conduction band and Γ point in the valence band ( Fig. 3c ). Thus, we expect enhancement in the band gap indirect emission when the carriers are excited in the band-nesting region. The PLE spectrum of the indirect peak (I) shows a distinct enhancement at the C absorption peak ( Fig. 3b ). On the other hand, the A emission peak shows relatively weaker enhancement in this energy range ( Fig. 3b ). 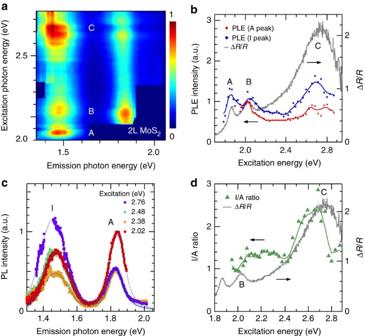Figure 3: PLE spectra of bilayer MoS2. (a,b) PLE intensity map and PLE spectra for bilayer MoS2. The PLE spectra are based on the integrated intensity of the A and I peak in the PL spectra at each excitation energy. The differential reflectance spectrum is also shown for comparison. The PLE spectrum of the A peak is normalized by the B exciton peak of the differential reflectance and the PLE of the I peak is multiplied by the same factor as the PLE spectrum of the A peak. (c) PL spectra collected with excitation energy of 2.02, 2.38, 2.48, 2.76 eV. (d) The ratio of integrated PL intensity between the I and A peak as a function of excited energy. The differential reflectance spectrum is also shown for comparison. Figure 3c,d show the evolution of the ratio of indirect (I) and direct (A) peaks. Similar results were obtained for bilayer WS 2 (see Supplementary Fig. 1 and Supplementary Note 1 for details). It may be noted that the band gap emission QY of bilayer samples was distinctly smaller (approximately four times) than that of monolayer samples (both mechanically exfoliated) for B peak excitation. In contrast, this ratio was only 2.6 for C peak excitation. These results further demonstrate that the photocarrier relaxation pathways and the radiative emission channels are uniquely related to band nesting. Figure 3: PLE spectra of bilayer MoS 2 . ( a , b ) PLE intensity map and PLE spectra for bilayer MoS 2 . The PLE spectra are based on the integrated intensity of the A and I peak in the PL spectra at each excitation energy. The differential reflectance spectrum is also shown for comparison. The PLE spectrum of the A peak is normalized by the B exciton peak of the differential reflectance and the PLE of the I peak is multiplied by the same factor as the PLE spectrum of the A peak. ( c ) PL spectra collected with excitation energy of 2.02, 2.38, 2.48, 2.76 eV. ( d ) The ratio of integrated PL intensity between the I and A peak as a function of excited energy. The differential reflectance spectrum is also shown for comparison. Full size image Carrier relaxation pathway The photocarriers relax through a series of phonon scattering, and are subject to the selection rules imposed by energy and momentum conservation. In the approximation of weakly interacting electron and hole, the electron–phonon scattering time is given by the Fermi golden rule [42] , [43] where | ψ i › and | ψ f › are the initial and final states with momentum k i and k f = k i − q and energies ε i and ε f . q is the scattering vector, is the interaction potential, and n B ( ħω , T ) is the Bose-Einstein distribution. The upper/lower elements correspond to phonon emission/absorption. 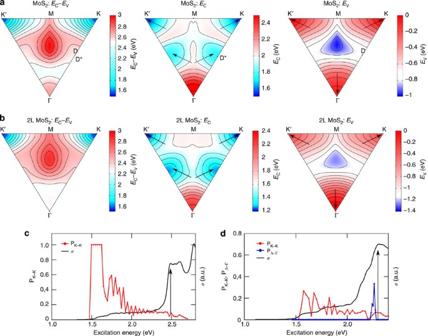Figure 4: Calculated energy landscape and optical spectra for monolayer and bilayer MoS2. (a,b) Energy map ofEc−Ev,EcandEvin the Brillouin zone for monolayer and bilayer MoS2. The arrows inEcandEvindicate possible relaxation pathways of carriers from the nesting region. (c,d) The fraction of electron–hole pairs that end the relaxation at the K point (PK−K, red curve) and the optical conductivity (σ, black curve) for monolayer and bilayer MoS2. Ford, the fraction of electron–hole pairs relaxing to Λ valley and Γ hill (PΛ−Γ) is also shown (blue plot). The arrows incanddindicate the position of the first peak due to band nesting. Figure 4a shows the potential contour of the nesting region in the first Brillouin zone along with the potential map of the conduction and the valence bands. We have defined these regions using the criteria | ∇ k ( E c − E v )| ≪ 1 eV/(2 π / a ) (ref. 25 ), where 2 π / a is the modulus of the reciprocal lattice vector, E c and E v are the energy in the unoccupied states in the conduction band (c) and the occupied states in the valence band (v), respectively. This region is highlighted in white in Fig. 4a . The arrows indicate the possible relaxation paths for electrons and holes after excitation in the nesting region. According to the DFT results, majority of the photocarriers are generated between Γ and Λ points. The electrons and holes are likely to relax into Λ and Γ points, respectively. Some photocarriers are also generated between Λ and K points where weak nesting is observed. Since the nesting between Λ and K points is relatively close to the K point, most of the photocarrier relax to the K points, giving rise to direct exciton emission. Note that monolayer WS 2 exhibits energy landscape similar to that of monolayer MoS 2 . (see Supplementary Fig. 2 and Supplementary Note 2 ). Similar potential maps are shown for bilayer MoS 2 ( Fig. 4b ). It can be seen that the nesting region is extended around the Γ point for bilayer compared with the case of monolayer. Figure 4: Calculated energy landscape and optical spectra for monolayer and bilayer MoS 2 . ( a , b ) Energy map of E c − E v , E c and E v in the Brillouin zone for monolayer and bilayer MoS 2 . The arrows in E c and E v indicate possible relaxation pathways of carriers from the nesting region. ( c , d ) The fraction of electron–hole pairs that end the relaxation at the K point (P K−K , red curve) and the optical conductivity ( σ , black curve) for monolayer and bilayer MoS 2 . For d , the fraction of electron–hole pairs relaxing to Λ valley and Γ hill (P Λ−Γ ) is also shown (blue plot). The arrows in c and d indicate the position of the first peak due to band nesting. Full size image We estimate the fraction of photocarriers reaching the conduction band minimum and valence band maximum at the K point after excitation at the nesting region for monolayer MoS 2 . Both acoustic and optical/homopolar phonons can intervene in the carrier relaxation, the former mainly through deformation potential interaction, and the latter mainly through Fröhlich interaction. In MoS 2 , the scattering rates have been calculated for both acoustic and optical phonons and were found to be comparable above the onset of optical phonon emission [44] . Further, both rates are approximately independent of q except for short wavelength acoustic phonons. Thus, we assume that all allowed phonon emission events are equally probable. The relaxation of the electron and hole were assumed to be independent and the process was stopped whenever the carrier was within a capture radius R (taken to be ~10 −4 2 π / a ) of a band extremum. The fraction of electron–hole pairs that end the relaxation at the K point is shown as a function of the excitation energy in Fig. 4c for monolayer MoS 2 . Between the energies corresponding to peaks A and B, the probability of electron–hole pairs relaxing to K is unity. However, this fraction becomes considerably lower at ~2 eV. This trend reproduces well the decrease of the relative QY at the C peak ( Fig. 2a ). From this energy onwards, the relaxation is mostly mediated by acoustic phonons. When the excitation energy is close to the C peak energy, a large fraction of the holes relax to the Γ point and electrons to the D* point (close to Λ). The energy of the first peak in the optical conductivity is due to nesting and is found at about 2.5 eV as indicated by the arrow in Fig. 4c . The population of relaxed carriers at the different stationary points of the Brillouin zone can be found in Supplementary Fig. 3 and Supplementary Note 2 . For bilayers MoS 2 , a similar trend is observed for the fraction of electron–hole pairs that reach the K point. The band nesting and corresponding divergence in the optical conductivity is observed at an excitation energy of ~2.4 eV. At this energy, rapid increase in the population of electrons and holes that relax to the Λ valley and Γ hill is observed. This trend explains the experimentally observed increase in the indirect emission intensity at the C peak absorption in bilayer MoS 2 ( Fig. 3b ). We summarize in Fig. 5 the possible relaxation pathways for monolayer and bilayer MX 2 when the excitation is in resonance with the band nesting energy. The system is initially excited from the ground state to the band nesting excited state (BN). A large fraction of these excited states relaxes to another excited state (Λ/Γ), which represents the state where electrons occupy the Λ valley and holes are at the Γ hill. Radiative recombination from this state competes unfavourably with the nonradiative decay ( ), which is a fast process (2–4 ps) (ref. 38 ), and intervalley scattering ( k iv ) to the lowest excited state (K/K), where both electrons and holes occupy the K point. Thus, only a small fraction of the initial excited states are transferred to the K/K state where radiative decay occurs with a moderate yield. In bilayer MX 2 , a sizeable fraction of the initial excited states decay to the Λ/Γ state where radiative indirect transition occurs with a modest yield. Note that this indirect emission does not compete with the intervalley scattering unlike the case of monolayer. Hot electron emission from the K/K state also occurs with non-negligible efficiency, partly due to intraband relaxation and intervalley scattering of hot carriers. 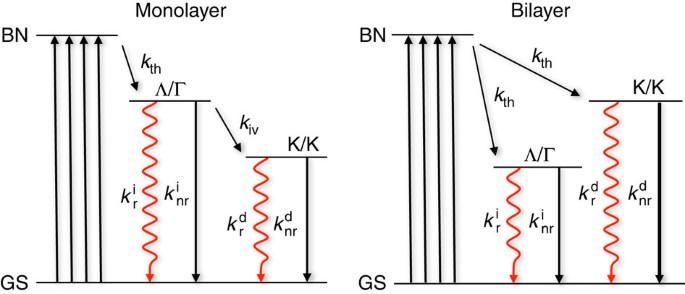Figure 5: Excitation and relaxation pathways for photocarriers. Energy diagram representing photocarrier relaxation channels in monolayer and bilayer MX2where the initial excitation is from the ground state (GS) to the band nesting (BN) energy. Nonraditive transition is indicated with a solid arrow. A rate constantkis associated with each transition. The subscripts indicate the types of transition: intravalley thermalization (th), intervalley scattering (iv), radiative (r) and nonradiative (nr). The superscripts (i) and (d) indicate indirect and direct transitions, respectively. Figure 5: Excitation and relaxation pathways for photocarriers. Energy diagram representing photocarrier relaxation channels in monolayer and bilayer MX 2 where the initial excitation is from the ground state (GS) to the band nesting (BN) energy. Nonraditive transition is indicated with a solid arrow. A rate constant k is associated with each transition. The subscripts indicate the types of transition: intravalley thermalization (th), intervalley scattering (iv), radiative (r) and nonradiative (nr). The superscripts (i) and (d) indicate indirect and direct transitions, respectively. Full size image The above qualitative model indicates that nonradiative decay rate k nr plays a crucial role in the carrier relaxation channels and emission intensity. It is known that k nr depends on the density of nonradiative decay centres, which may come from the trap states of the substrate, surface impurities, and intrinsic defects of the material [38] , [41] . We investigated the effects of nonradiative decay channels by arbitrarily reducing k nr by using the hexagonal boron nitride as the substrate. We found that this leads not only to the overall enhancement in the PL intensity but also slight increase in the relative QY at the C peak excitation, supporting the validity of the above model (see Supplementary Fig. 4 and Supplementary Note 3 for details). Strong light-matter interaction in semiconducting 2D TMDs is a remarkable feature that makes these materials attractive for their use in optoelectronics. Band nesting plays a crucial role in the spontaneous separation of electron–hole pairs in the k -space and temporary suppression of their relaxation to the fundamental band edge. Our findings provide insight into the unique dynamics of photocarrier relaxation pathways and motivate studies on the hot electron behaviours in 2D materials and their potential for efficient hot carrier collection devices. Sample preparation The samples used in this study were monolayer (and bilayer) MoS 2 , MoSe 2 , WS 2 and WSe 2 crystalline flakes. For MoS 2 , we studied mechanically exfoliated flakes as well as chemical vapour deposition-grown samples (see Supplementary Fig. 4 and Supplementary Note 3 for details). Monolayer MoS 2 on quartz substrate was directly grown by chemical vapour deposition. Single bulk crystals of MoSe 2 , WS 2 and WSe 2 were grown by chemical vapour transport using iodine as the transport agent. The crystals were mechanically exfoliated and deposited on quartz substrates. The number of layers was verified by PL, differential reflectance, Raman spectra and atomic force microscopy (see Supplementary Figs 5 and 6 for details). Optical measurements The measurements of differential reflectance were performed using a tungsten halogen lamp. The micro-PL spectra under a back scattering geometry were obtained by monochromator and a super-continuum light as an excitation source coupled to a tunable laser filter. The excitation intensities for PL and PLE measurements were kept below 10 μW in which the effect of optical non-linearity is negligible (see Supplementary Fig. 7 and Supplementary Note 4 for details). The measured spectral data were corrected for variations in the detection sensitivity with the correction factors obtained by using a standard tungsten halogen lamp. The differential reflectance is defined as ( R S+Q − R Q )/ R Q where R S+Q and R Q are the reflected light intensities from the quartz substrate with and without the material, respectively [6] , [34] , [45] . Theoretical calculations We performed a series of DFT calculations for the semiconductor TMDs family using the open source code QUANTUM ESPRESSO [46] . The JDOS, the dielectric permittivity and the optical conductivity were calculated using a modified version of the epsilon programme of the QUANTUM ESPRESSO distribution to account for full relativistic calculations. We calculated the optical conductivity directly from the band structure [46] . We used norm-conserving, fully relativistic pseudopotentials with nonlinear core-correction and spin-orbit information to describe the ion cores. The pseudopotentials used were either obtained from the QUANTUM ESPRESSO distribution or produced using the ATOMIC code by A. Dal Corso. The exchange correlation energy was described by the generalized gradient approximation, in the scheme proposed by Perdew, Burke and Ernzerhof [47] . The integrations over the Brillouin zone were performed using a scheme proposed by Monkhorst–Pack [48] for all calculations. Single-layer samples were modelled in a slab geometry by including a vacuum region of 45 bohr in the direction perpendicular to the surface. A grid of 16 × 16 × 1 k points was used to sample the Brillouin zone. The energy cutoff was 50 Ry. The atomic positions were optimized using the Broyden–Fletcher–Goldfarb–Shanno method for the symmetric structure. The lattice parameter a was determined by minimization of the total energy. A Gaussian broadening of 0.05-eV width was applied in the optical conductivity. It is well known that generalized gradient approximation underestimates the band-gap [29] , and hence the optical conductivity shows the peaks displaced towards lower energies relative to actual experiments. However, their shapes and intensities are expected to be correct. How to cite this article: Kozawa, D. et al. Photocarrier relaxation pathway in two-dimensional semiconducting transition metal dichalcogenides. Nat. Commun. 5:4543 doi: 10.1038/ncomms5543 (2014).